Surface-wetting effects on the liquid–liquid transition of a single-component molecular liquid Even a single-component liquid may have more than two liquid states. The transition between them is called a 'liquid–liquid transition' (LLT). Such LLTs have recently attracted considerable attention mainly because of the fundamental interest in the physical origin of this counter-intuitive phenomenon. In this study, we report the first observation of wetting effects on LLT for a molecular liquid, triphenyl phosphite. We find a transition from partial to complete wetting for nucleation-growth-type LLT when approaching the spinodal temperature of LLT. Some features unique to LLT are also revealed, reflecting for example the non-conserved nature of its order parameter. We also find that the wetting behaviour is not induced by dispersion forces, but by weak hydrogen bonding to a solid substrate, implying its important role in the LLT itself. Using wetting effects may open a new possibility to control kinetics and spatial patterns of nucleation-growth-type LLT. Surface-wetting effects [1] are known to have significant influences on pattern evolution, accompanied by phase transitions such as crystallization, phase separation and vapour–liquid transitions [2] , [3] , [4] , [5] , [6] . For example, nucleation and growth (NG) of a new phase, which has a lower free energy than a metastable phase, is ubiquitous in a variety of first-order phase transitions. This process of the emergence of a new phase has to overcome a free-energy barrier associated with the formation of an interface separating the new and old phase. If there is a mechanism lowering the barrier, the process should be significantly accelerated. Heterogeneous nucleation is one of such examples. If a third solid material friendly enough to a new phase is in contact with a metastable liquid, nucleation of the new phase preferentially takes place on the solid material. The key factor controlling this process is the wettability of the new phase on the solid material. There are a number of studies on both homogeneous and heterogeneous nucleation phenomena that span over a century. In particular, the initial stage of nucleation has continued to attract much attention from the fundamental viewpoint [7] , [8] , [9] . From the applications viewpoint, on the other hand, heterogeneous nucleation is widely used as a catalyst for producing high-quality single crystals of, for example, semiconductors and proteins, which allows us to avoid spontaneous homogeneous nucleation in bulk. Recently, chemical and topological control of wettability has become key to the design of micro- and nanoscale pattern formation processes at surfaces and in thin films, which is crucial for nanotechnology (see for example refs. 4 , 10 ). Surface-wetting effects have so far been intensively studied for phase transitions such as crystallization, vapour–liquid phase transition and phase separation of a binary mixture [1] , [2] , [3] , [4] , [5] , [6] . In this study, we focus our attention on a novel type of first-order phase transition: 'liquid–liquid transition' (LLT) in a single-component liquid. This phenomenon, which is contradictory to the common belief that there is only one liquid state for a single-component liquid, has attracted considerable attention because of its counter-intuitive nature. Recently, there have been growing experimental and numerical pieces of evidence that even a single-component liquid can have more than two liquid states and there is a first-order phase transition between them [11] , [12] , [13] , [14] , [15] , [16] . However, direct experimental evidence is rather limited and often disputed. For example, a structural transition in phosphorus [14] accompanies a large volume change of 40%. This volume change is too large for a first-order transition between two liquid states. The transition is now regarded as a 'supercritical fluid'–liquid transition rather than an LLT [17] . In the case of yttria-alumina [13] , [16] , there are still on-going debates on the composition range over which this phenomenon occurs and the experimental conditions required to produce the effect [18] . Furthermore, a recent report of the direct observation of a first-order liquid–liquid phase transition by Greaves et al . [19] has recently been questioned by Barnes et al . [20] Recently, we found experimental evidence for the existence of LLT in two molecular liquids, triphenyl phosphite (TPP) [21] , [22] and n-butanol [23] , at ambient pressure, following the finding of the so-called glacial state in this material [24] . This phenomenon was claimed by Hedoux et al . [25] to be induced by the formation of microcrystallites. Some researchers suspect that it may be a phase separation into a TPP-rich and an impurity-rich phase, as TPP molecules are known to decompose under the presence of water because of ester hydrolysis. However, we found the following evidence, which cannot be explained by such scenarios. We revealed that LLT proceeds through two types of kinetics: NG and spinodal decomposition (SD) [22] , [23] . For NG-type LLT, the liquid II phase is nucleated as droplets and their size grow linearly with time. For SD-type LLT, on the other hand, liquid I transforms into liquid II continuously, accompanying spatial fluctuations of the order parameter. At a low temperature, in which we see SD-type LLT, we confirmed that there is no indication of the presence of microcrystallites [21] , [22] . Furthermore, we also found the criticality associated with LLT: critical divergence of the correlation length of the order parameter fluctuations [22] . The kinetics is found to be well described by our two-order-parameter model of LLT [26] , which regards LLT as a gas–liquid-like cooperative ordering of a non-conserved scalar order parameter S , which may be the fraction of locally favoured structures. The non-conserved nature of the order parameter also shows that the phenomenon is not explained by phase separation. Although LLT is a counter-intuitive phenomenon, it can be naturally explained by assuming that an extra scalar order parameter is necessary to specify a liquid state, in addition to density ρ [26] . We proposed that it is the number density of a locally favoured structure S , as mentioned above. Then LLT can be regarded as a gas–liquid-like first-order phase transition between a gas (dilute) state and a liquid (dense) state of locally favoured structures. As locally favoured structures can be created and annihilated rather independently, the order parameter S should be of a non-conserved nature, unlike density ρ . This explains why liquid I completely transforms into liquid II (without coexistence), unlike phase separation. In this scenario, a liquid can sequentially have two first-order transitions, besides a liquid–solid transition/gas–liquid and LLT. The former is dominated by ρ , whereas the latter is dominated by S . LLT generally accompanies the change in physical and chemical properties of a liquid. For example, the density and refractive index of liquid I are lower than those of liquid II for TPP [21] , [24] and n-butanol [23] . The dielectric constant of liquid II is lower than that of liquid I [27] . Liquid I is a viscous liquid, whereas liquid II is a glassy amorphous solid. Furthermore, fragility, which characterizes how steeply viscosity increases when approaching T g , is larger for liquid I than for liquid II [21] , [28] . Liquid I of TPP is a typical fragile liquid, but becomes stronger as LLT proceeds, and the final liquid II is as strong as B 2 O 3 . Very recently, we also found that miscibility with other liquids is different between liquid I and II [29] . These facts indicate that liquid properties such as density, refractive index, viscosity, fragility and miscibility strongly depend on the order parameter S . This suggests that the wettability to a solid substrate may also be different between liquid I and II. However, wetting effects on LLT have not been investigated so far. In this article, we study how wetting effects affect the pattern evolution of LLT in the presence of a solid substrate. This provides a unique opportunity to investigate wetting effects on a first-order phase transition governed by a non-conserved order parameter in a liquid state. We show that pattern evolution and kinetics of NG-type LLT can be controlled by surface-wetting effects. This has an important implication for the future application of LLT. We also find a partial-to-complete wetting transition when approaching the mean-field spinodal temperature T SD . This critical-point wetting behaviour [2] provides further strong evidence for the criticality associated with LLT. This further supports a conclusion that the phenomenon observed in TPP is truly 'LLT'. Wetting effects on the pattern evolution of LLT To study wetting effects on LLT, we used various dielectric and metallic solids as a substrate, which is in contact with TPP during LLT (see Methods section). We note that NG-type LLT occurs below the binodal temperature T BN =232 K, whereas SD-type LLT occurs below the spinodal temperature T SD =215.5 K [21] . We first describe NG-type LLT ( T SD < T < T BN ) for a case of complete wetting. 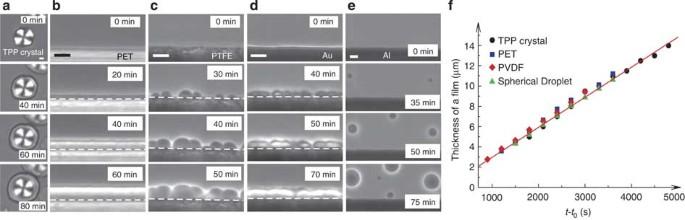Figure 1: Heterogeneous nucleation of liquid II on various solid surfaces at 220 K. (a) Time evolution of LLT in the presence of a TPP crystal, which was observed with polarizing microscopy under the crossed Nicols condition. At the beginning (0 min), we observe only the TPP crystalline spherulite with the Maltese cross pattern. Thereafter, the layer of liquid II, which has no birefringence, is formed on the surface of the TPP spherulite (40 min) and its thickness linearly grows with time (60, 80 min) (seef). (b) Time evolution of LLT in the presence of a PET surface. In this case, LLT proceeds while forming a thin film of liquid II, which also grows linearly with time (seef): compete wetting. White dashed lines indicate the location of the surface. (c,d) Time evolution of LLT in the presence of PTFE (c) and gold (d) surface. Nuclei of liquid II are preferentially formed on the substrates with a finite contact angle (θ≤90°): partial wetting. (e) Time evolution of LLT in the presence of an aluminium surface. Nuclei of liquid II do not have any contact to the aluminium surface and normal NG-type droplet growth in bulk was observed: non-wetting. The scale bars correspond to 10 μm. (f) Growth kinetics of a complete wetting layer of liquid II. Time evolution of the thickness of the wetting layer (left axis) formed on a TPP crystal (a), PET (b) and PVDF (Fig. 2b) surface, together with the radius of a droplet of liquid II (right axis). Timetis shifted by birth timet0. Temperature was 220 K. All data can be well fitted by linear functions, indicating the same growth rate irrespective of the substrate materials. The growth rate of the wetting layer is estimated as 2.95±0.15 nm s−1. Figure 1a shows pattern evolution during heterogeneous nucleation on a TPP crystalline surface at 220 K. Before the temperature quench ( t <0), the spherulite of the TPP crystal with optical birefringence (manifested by the Maltese cross) grows in the homogeneous liquid I at 235 K. Immediately after a temperature quench to 220 K, LLT is initiated and the layer of liquid II is formed preferentially on the surface of the TPP crystalline spherulite ( t =40 min). Thereafter, its thickness linearly grows with time ( t =60 min, 80 min) (see below). Figure 1b shows the process of heterogeneous nucleation of liquid II on a poly(ethylene terephthalate) (PET) surface at 220 K. Unlike usual NG-type transformations, LLT proceeds while accompanying the formation of a thin film of liquid II on the solid surface for both TPP crystal and PET case: complete wetting. In these cases, nucleation occurs preferentially on solid surfaces. Figure 1c,d show the processes of heterogeneous nucleation of liquid II on poly(tetrafluoroethylene) (PTFE) and gold surfaces at 220 K, respectively. In these cases, we observe partial wetting behaviour. A contact angle is estimated to be about 74° for PTFE and 62° for gold. We can see that the nucleation rate is much higher on the surface than in bulk. This behaviour is consistent with the typical heterogeneous nucleation behaviour known for other types of phase transitions such as crystallization and phase separation [11] . Partial wetting behaviour is also observed for poly(ethylene naphthalate), poly(imide) and poly(vinylidene difluoride) (PVDF) surfaces, as shown in Fig. 2 . Figure 1e shows pattern evolution during LLT on an aluminium surface. We observe that nuclei of liquid II do not have any contact with the aluminium surface, and NG-type LLT occurs solely in bulk (not on the surface). This is characteristic of non-wetting behaviour. In other words, the wettability of liquid I to the substrate is higher than that of liquid II. Such behaviour is also observed for poly(ethylene) (PE) (see Fig. 2d ). Figure 1: Heterogeneous nucleation of liquid II on various solid surfaces at 220 K. ( a ) Time evolution of LLT in the presence of a TPP crystal, which was observed with polarizing microscopy under the crossed Nicols condition. At the beginning (0 min), we observe only the TPP crystalline spherulite with the Maltese cross pattern. Thereafter, the layer of liquid II, which has no birefringence, is formed on the surface of the TPP spherulite (40 min) and its thickness linearly grows with time (60, 80 min) (see f ). ( b ) Time evolution of LLT in the presence of a PET surface. In this case, LLT proceeds while forming a thin film of liquid II, which also grows linearly with time (see f ): compete wetting. White dashed lines indicate the location of the surface. ( c , d ) Time evolution of LLT in the presence of PTFE ( c ) and gold ( d ) surface. Nuclei of liquid II are preferentially formed on the substrates with a finite contact angle ( θ ≤90°): partial wetting. ( e ) Time evolution of LLT in the presence of an aluminium surface. Nuclei of liquid II do not have any contact to the aluminium surface and normal NG-type droplet growth in bulk was observed: non-wetting. The scale bars correspond to 10 μm. ( f ) Growth kinetics of a complete wetting layer of liquid II. Time evolution of the thickness of the wetting layer (left axis) formed on a TPP crystal ( a ), PET ( b ) and PVDF ( Fig. 2b ) surface, together with the radius of a droplet of liquid II (right axis). Time t is shifted by birth time t 0 . Temperature was 220 K. All data can be well fitted by linear functions, indicating the same growth rate irrespective of the substrate materials. The growth rate of the wetting layer is estimated as 2.95±0.15 nm s −1 . 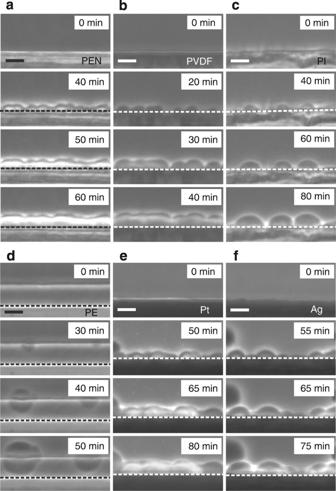Figure 2: Heterogeneous nucleation during LLT at 220 K from the surface. (a) PEN (poly(ethylene naphthalate)), (b) PVDF, (c) PI, (d) PE, (e) platinum, (f) silver. Dashed lines indicate the surface of substrates. Ford, a very thin film of PE extends along the glass plate beyond the dashed line (whitish horizontal line), but it does not affect the nucleation behaviour. The scale bars correspond to 10 μm. Full size image Figure 2: Heterogeneous nucleation during LLT at 220 K from the surface. ( a ) PEN (poly(ethylene naphthalate)), ( b ) PVDF, ( c ) PI, ( d ) PE, ( e ) platinum, ( f ) silver. Dashed lines indicate the surface of substrates. For d , a very thin film of PE extends along the glass plate beyond the dashed line (whitish horizontal line), but it does not affect the nucleation behaviour. The scale bars correspond to 10 μm. Full size image Here, we show the growth kinetics of wetting layers for three substrates exhibiting complete wetting, TPP crystal, PET and PVDF, together with the growth of an isolated nucleus of liquid II, in Fig. 1f . In all the cases, domains grow linearly with the same growth speed: V =2.95±0.15 nm s −1 . This linear growth is consistent with the wetting layer growth in a metastable state for a system of a non-conserved order parameter [30] . The insensitivity of the growth rate on substrates indicates that the growth speed perpendicular to a substrate does not depend on the type of substrate, as expected. We note that according to the classical nucleation theory [31] , growth velocity V is given by , where k is a constant, k B is Boltzmann's constant, τ t is the characteristic time of material transport, ν m is a volume per molecule and δμ is the chemical potential difference per unit volume between liquid I and II. This indicates that V should not depend on substrates for complete wetting. For a binary liquid mixture, for example, Bonn et al . [32] observed pronounced hysteresis effects on a wetting process when the equilibrium film thickness is large. They also reported a power law growth of the wetting layer after the nucleation process, in agreement with a diffusion-limited growth mechanism [33] . As we do not have access to the very early stage of wetting, we cannot provide any information on the process of nucleation of a wetting layer at this moment. This deserves future investigation. On the layer growth kinetics, on the other hand, there should be a crucial difference between phase separation and LLT (see the above), reflecting whether the order parameter is conserved. A transition between partial and complete wetting We also find a transition from partial to complete wetting when approaching T SD . 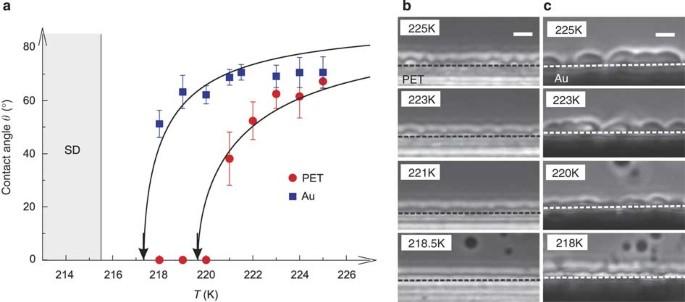Figure 3: Temperature dependence of the wetting behaviour of liquid II nearTSD. (a) Temperature dependence ofθfor PET and gold substrates. Error bars indicate the variance of a number of (about 20) independent measurements of the wetting angle. Curves are the results of the fitting of the following function:θ=cos−1(At−1), whereA=ΔγS/γ0. For PET,A=0.0193±0.0007 and for gold,A=0.0085±0.0007. The wetting transition temperatureTwis estimated asTw=219.6 K for the PET substrate.θfor the gold substrate also decreases to zero while approachingTSD. For the gold substrate,Twis estimated as 217 K, slightly aboveTSD. Phase-contrast microscopy images of the wetting behaviour of liquid II at various temperatures are shown for the PET (b) and gold substrate (c). Scale bars correspond to 10 μm. Figure 3 shows the temperature ( T ) dependence of the contact angle θ , together with microscopy images for PET and gold substrates. For a PET surface, a partial-to-complete wetting transition takes place around 220 K. For gold, on the other hand, θ tends to decrease toward zero near T SD on cooling. These results are reminiscent of 'critical-point wetting', which is universally observed near a critical point of a gas–liquid transition or phase separation of a binary liquid mixture [2] . The contact angle θ should follow Young's law: θ =cos −1 [( γ SI − γ SII )/ γ ], where γ SI and γ SII are the contact energy per unit area of a solid substrate to liquid I and II, respectively, and γ is the interfacial tension between liquid I and II. Thus, the partial-to-complete wetting transition observed should be due to the vanishing interfacial tension γ toward T SD , reflecting the diverging correlation length ξ of an order parameter. For LLT of TPP, we confirmed the mean-field nature of the criticality [22] : ξ = ξ 0 t −1/2 , where t =( T − T SD )/ T SD is the reduced temperature. According to the mean-field theory, γ = γ 0 t 3/2 and γ SI − γ SII =Δ γ S t 1/2 . Thus, we have a prediction for the T -dependence of θ : θ =cos −1 [Δ γ S / γ 0 t −1 ]. This relation reasonably explains the experimental results (see Fig. 3 ). This critical nature of wetting behaviour in LLT strongly suggests that T SD has a role as a hidden critical point of the system [21] , [22] . At this stage, however, we cannot draw a definite conclusion on the details of this transition, such as its order and the critical exponent, as our measurement of θ is a bit far from T SD because of experimental difficulties. Here, it may be worth noting that such critical-point wetting is generally observed rather far from a critical point [6] , [34] , contrary to what its name suggests. Figure 3: Temperature dependence of the wetting behaviour of liquid II near T SD . ( a ) Temperature dependence of θ for PET and gold substrates. Error bars indicate the variance of a number of (about 20) independent measurements of the wetting angle. Curves are the results of the fitting of the following function: θ =cos −1 ( At −1 ), where A =Δ γ S / γ 0 . For PET, A =0.0193±0.0007 and for gold, A =0.0085±0.0007. The wetting transition temperature T w is estimated as T w =219.6 K for the PET substrate. θ for the gold substrate also decreases to zero while approaching T SD . For the gold substrate, T w is estimated as 217 K, slightly above T SD . Phase-contrast microscopy images of the wetting behaviour of liquid II at various temperatures are shown for the PET ( b ) and gold substrate ( c ). Scale bars correspond to 10 μm. Full size image Confinement effects on the kinetics of NG-type LLT Surface-assisted nucleation can significantly accelerate NG-type LLT in a thin-film geometry. 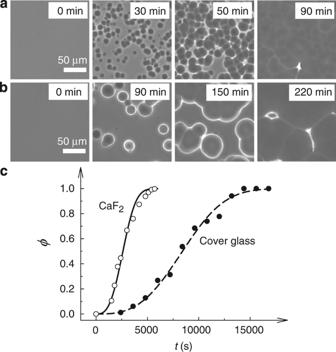Figure 4: Effects of surface wettability on the kinetics of NG-type LLT confined in a quasi two-dimensional geometry. (a) NG-type LLT observed using phase-contrast microscopy atT=220 K in a TPP sample (thickness=10 μm) sandwiched by two calcium fluoride plates, which exhibit partial wetting behaviour. The scale bar corresponds to 50 μm. (b) The same asaexcept that a sample is sandwiched by two cover glasses that exhibit non-wetting behaviour. (c) Time evolution of the volume (area) fraction φ of liquid II for bothaandb. We can see that the nucleation frequency is much higher for the substrate with stronger wettability (a), which leads to the faster transformation of liquid I to liquid II fora. The curves are the fitting of the Avrami–Kolmogolov equation φ (t)=1−exp (−Ktn) to the data, whereK=(π/3)JV2is the Avrami coefficient andnis the Avrami exponent. Here, we obtainn=3, which means that nuclei appear homogeneously in two-dimension (although heterogeneous along the thickness direction) and grow isotropically. The values ofK, growth velocityVand nucleation rateJestimated from the above analysis areK=3.88×10−11s−3,V=3.29 nm s−1andJ=3.42×106s−1 m−2for the case of calcium fluoride substrates, whereasK=1.16×10−11s−3,V=3.00 nm s−1andJ=1.24×106s−1 m−2for the case of cover glasses. Figure 4 shows such an example. We can clearly see that the nucleation rate of liquid II is much higher for the TPP confined between two calcium fluoride plates exhibiting partial wetting than for that confined between two non-wetting cover glasses. The nucleation frequency estimated from the Avrami analysis was about three times higher for the former than for the latter (see the caption of Fig. 4c ). This is because of the surface-induced nucleation of liquid II. This indicates that we can accelerate the kinetics of NG-type LLT itself significantly by spatially confining TPP into a material wettable to liquid II. Figure 4: Effects of surface wettability on the kinetics of NG-type LLT confined in a quasi two-dimensional geometry. ( a ) NG-type LLT observed using phase-contrast microscopy at T =220 K in a TPP sample (thickness=10 μm) sandwiched by two calcium fluoride plates, which exhibit partial wetting behaviour. The scale bar corresponds to 50 μm. ( b ) The same as a except that a sample is sandwiched by two cover glasses that exhibit non-wetting behaviour. ( c ) Time evolution of the volume (area) fraction φ of liquid II for both a and b . We can see that the nucleation frequency is much higher for the substrate with stronger wettability ( a ), which leads to the faster transformation of liquid I to liquid II for a . The curves are the fitting of the Avrami–Kolmogolov equation φ ( t )=1−exp (− Kt n ) to the data, where K =( π /3) JV 2 is the Avrami coefficient and n is the Avrami exponent. Here, we obtain n =3, which means that nuclei appear homogeneously in two-dimension (although heterogeneous along the thickness direction) and grow isotropically. The values of K , growth velocity V and nucleation rate J estimated from the above analysis are K =3.88×10 −11 s −3 , V =3.29 nm s −1 and J =3.42×10 6 s −1 m−2 for the case of calcium fluoride substrates, whereas K =1.16×10 −11 s −3 , V =3.00 nm s −1 and J =1.24×10 6 s −1 m−2 for the case of cover glasses. Full size image Wetting effects on SD-type LLT Next we mention surface-wetting effects on SD-type LLT. 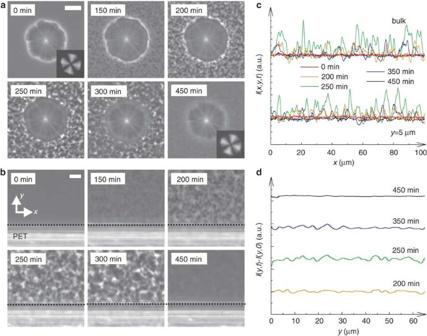Figure 5: Wetting behaviour for SD-type LLT. (a) Pattern evolution during SD-type LLT in the presence of a TPP crystal (formed at 235 K), which is observed with phase-contrast microscopy at 213 K (<TSD). Insets show the images observed with polarizing microscopy under a crossed Nicols condition. The white bar corresponds to 20 μm. (b) Pattern evolution during SD-type LLT in the presence of a PET surface, which is observed with phase-contrast microscopy at 213 K. The black dotted lines indicate the location of the surface of PET. The white bar corresponds to 10 μm. For both cases ofaandb, the amplitude of the order parameter fluctuations increases with time initially, but later decays with time, and finally becomes a homogeneous liquid II state21,22. The characteristic lengthscale of fluctuations keeps increasing with time. We cannot see any indication of surface-wetting effects on LLT at least on a macroscopic level. (c) The intensity profileI(x,y,t) obtained from the micrographs inb, along thexdirection aty=5 μm (near surface) andy=100 μm (in bulk). The PET surface is located aty=0 μm. (d) The intensity profile in b along theydirection, which is averaged along thexdirection over 100 μm. Here(L: the length alongx). We cannot see any distinct density profile near the surface (y=0 μm) (for example, a density wave and/or a wetting layer), suggesting the absence of distinct surface-wetting effects. Figure 5a,b show a pattern evolution process of SD-type transformation in the presence of a TPP crystal and a PET surface at 213 K, respectively. We already observe for NG-type LLT that liquid II completely wets both TPP crystal and PET surface. For SD-type LLT, however, we do not observe any indication of wetting effects on pattern evolution for both surfaces: the wetting layer is absent, at least on a macroscopic length scale. In Fig. 5c , we show the intensity (or density) profile obtained from the images, along the x direction at y =5 μm and y =100 μm (bulk) from the PET surface. In Fig. 5d , on the other hand, we show the intensity profiles along the y direction, which are averaged along the x direction over 100 μm to suppress the amplitude of intensity fluctuations due to spatial fluctuations of the order parameter S . We can observe the growth of the fluctuation amplitude (200, 250 min) and its coarsening (350, 450 min) during LLT, both at y =5 μm and in bulk (see Fig. 5c ), which is characteristic of typical SD-type LLT [21] , [22] . However, we observe neither kinetic acceleration of LLT nor wetting layer formation of liquid II near the surface (see Fig. 5d ). Figure 5: Wetting behaviour for SD-type LLT. ( a ) Pattern evolution during SD-type LLT in the presence of a TPP crystal (formed at 235 K), which is observed with phase-contrast microscopy at 213 K (< T SD ). Insets show the images observed with polarizing microscopy under a crossed Nicols condition. The white bar corresponds to 20 μm. ( b ) Pattern evolution during SD-type LLT in the presence of a PET surface, which is observed with phase-contrast microscopy at 213 K. The black dotted lines indicate the location of the surface of PET. The white bar corresponds to 10 μm. For both cases of a and b , the amplitude of the order parameter fluctuations increases with time initially, but later decays with time, and finally becomes a homogeneous liquid II state [21] , [22] . The characteristic lengthscale of fluctuations keeps increasing with time. We cannot see any indication of surface-wetting effects on LLT at least on a macroscopic level. ( c ) The intensity profile I ( x , y , t ) obtained from the micrographs in b , along the x direction at y =5 μm (near surface) and y =100 μm (in bulk). The PET surface is located at y =0 μm. ( d ) The intensity profile in b along the y direction, which is averaged along the x direction over 100 μm. Here ( L : the length along x ). We cannot see any distinct density profile near the surface ( y =0 μm) (for example, a density wave and/or a wetting layer), suggesting the absence of distinct surface-wetting effects. Full size image Now we discuss a key physical factor controlling the wettability of liquid II to a solid surface. First we check the role of the dispersion force, which is known to have a crucial role in usual wetting phenomena [1] , [6] , [35] . To do so, we calculate a non-retarded Hamaker constant H between liquid II and a dielectric solid surface on the basis of the Lifshitz theory [35] (See Methods for details). Table 1 shows the values of H at 220 K estimated in this manner, together with the measured θ , which is the angle between the solid surface and the surface of liquid II, for dielectric solid substrates. Table 2 , on the other hand, lists parameters used for the estimation based on the Drude model [35] and H , together with θ measured at 220 K for metallic solid substrates (see Methods for the details). Tables 1 and 2 clearly tell us that there is no correlation between H and θ for both dielectric and metallic solid surfaces. This suggests that van der Waals interactions are not responsible for the surface-wetting phenomena observed for LLT and the key factor dominating wettability may be a specific interaction of microscopic nature. Table 1 Included in this table are the dielectric constant ϵ 0 , the refractive index n , the measured contact angle θ and the non-retarded Hamaker constant H between liquid II and the following dielectric solids immersed in liquid I: TPP crystal, PET, PEN, PI, PVDF, PTFE, PE and calcium fluoride. Full size table Table 2 Included in this table are the plasma frequency ν p and the damping frequency γ for the Drude model, the measured contact angle θ and the non-retarded Hamaker constant H between liquid II and the following metallic substrates immersed in liquid I: gold, platinum, silver, aluminium. Full size table There are many candidates for forces responsible for the wetting phenomena observed, such as short-range forces, besides the dispersion forces [6] . Here, we consider an electron acceptor–donor interaction [36] as a natural candidate for specific interactions in our systems. We note that there is a considerable difference in wetting behaviour between PVDF, PTFE and PE surfaces, despite the fact that they have similar basic molecular structures. Although the values of H for PVDF and PTFE are negative and smaller than that for PE, liquid II shows partial wetting to PVDF and PTFE but does not wet PE at all at 220 K. Furthermore, despite a negative value of H , liquid II shows complete wetting to PET at 220 K. For metallic surfaces, we found that aluminium, which is not categorized as a transition metal, shows non-wetting behaviour at 220 K, whereas the other metals, which are categorized as transition metals, exhibit partial wetting behaviour. Recently, the importance of weak hydrogen bonding to transition metals has been gradually accepted [37] . We propose the following mechanism for the wetting behaviour observed: Atoms of high electronegativity in a substrate induce weak hydrogen bonding to TPP molecules. For example, fluorine (F) and oxygen (O) atoms in dielectric substrates induce C–F ⋯ …H–C and C=O…H–C, whereas electron-rich transition metal (M) atoms induce M…H–C and M…P–O. It is such weak hydrogen bonding that promotes nucleation of liquid II on the surfaces. This scenario is consistent with recent experimental and numerical studies, which suggest the importance of intermolecular weak hydrogen bonding in the formation of liquid II of TPP [38] , [39] . It is also known that the existence of surfaces having direct interactions to molecules leads to surface-induced self-assembly of molecules [40] . From Tables 1 and 2 , we can also see that liquid II does not wet surfaces having only van der Waals interactions with TPP (PE, aluminium). All these indicate that the wetting behaviour of liquid II during LLT is dominated by the ability of a substrate to enhance the formation of weak hydrogen bonding. This has a further important implication on the very origin of LLT in TPP: Locally favoured structures, the number density S of which may be the order parameter governing LLT [26] , may also be induced by weak hydrogen bonding between TPP molecules. The relevance of the above wetting mechanism may be directly confirmed by using surface-sensitive spectroscopic methods such as surface-enhanced Raman spectroscopy. Such a short-range nature of the surface field is also interesting in the context of critical-point wetting. Wetting transition under a short-range force has attracted considerable attention [6] , [41] , [42] , [43] , as its upper critical dimension d u , above which the mean-field theory is valid, becomes three ( d u =3). Most examples of wetting transitions observed are of first order as they are influenced by long-range van der Waals forces in usual experimental situations. Recently, Ross et al . [44] successfully observed a critical wetting transition under short-range force near a critical point. However, such a case is still rare. The wetting transition of LLT may provide us not only with an ideal example of wetting under a short-range force but also with valuable information on the criticality of LLT. Next, we consider why surface-wetting effects have little influence on SD-type LLT (see Fig. 5 ). It is known that for phase separation of a binary mixture, the kinetics of SD is seriously influenced by surface wettability, due to formation of a composition wave near a surface and the rapid hydrodynamic growth of a wetting layer. This is particularly the case for phase separation of binary fluid mixtures [5] , [45] . For example, hydrodynamic flow induced by the pressure gradient from bulk to a surface significantly accelerates bicontinuous SD, which leads to the t -linear growth of the wetting layer on a substrate [5] , [46] , [47] . However, such behaviour is not observed for SD-type LLT, at least on a macroscopic lengthscale. According to our two-order-parameter model of LLT, LLT is primarily driven by the ordering of a non-conserved order parameter, S , and the density ρ changes only through its coupling to S . The validity of such a model has been checked by comparing simulations with experimental results [48] . For a system with a non-conserved order parameter under a short-range force, a wetting layer is predicted to grow as log t in an unstable region [30] . This extremely slow coarsening may explain why we cannot observe the growth of a wetting layer on a macroscopic lengthscale. Fast-growing fluctuations in bulk overwhelm a slowly growing wetting layer. For NG-type LLT, on the other hand, the slowness of nucleation of liquid II in bulk and the fast t -linear growth of a wetting domain (see Fig. 1f ) make the wetting effects distinct. Furthermore, the non-conserved nature allows a 'local' change of the order parameter, which leads to the absence of a surface-induced oscillation of the order parameter along the direction perpendicular to a surface for SD-type LLT (see Fig. 5d ). This is markedly different from the situation of a binary mixture [4] , in which a surface-induced composition wave is produced, as the increase in concentration near the surface must accompany its decrease nearby to satisfy the material conservation. In addition, a sharp interface is never formed for SD-type LLT, also because of the non-conserved nature of the order parameter [21] , [22] , which makes interface-tension-driven flow very weak and inactive: local order parameter evolution dominates the process. All these support the non-conserved nature of the order parameter of LLT. In pure TPP, the system becomes more glassy during SD-type LLT, which also weakens the flow. In relation to this, it is worth noting that we also confirm the absence of surface-wetting effects on SD-type LLT even for a TPP/toluene (75/25) mixture in the presence of a PET substrate (see Fig. 6 ). In this case, the final liquid II remains a viscous liquid, unlike pure TPP, which becomes a glassy amorphous solid state of liquid II after LLT [29] . These confirm the absence of surface-wetting effects on SD-type LLT and the above explanation. 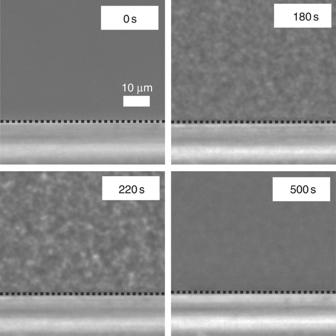Figure 6: SD-type LLT in a TPP/toluene (75/25) mixture observed with phase-contrast microscopy near a PET film. Even though PET is a substrate inducing complete wetting for NG-type LLT, we do not see any indication of either the density wave or the formation of a wetting layer. This indicates that surface-wetting effects are inactive for SD-type LLT. Black dashed lines indicate the surface of the PET film. Figure 6: SD-type LLT in a TPP/toluene (75/25) mixture observed with phase-contrast microscopy near a PET film. Even though PET is a substrate inducing complete wetting for NG-type LLT, we do not see any indication of either the density wave or the formation of a wetting layer. This indicates that surface-wetting effects are inactive for SD-type LLT. Black dashed lines indicate the surface of the PET film. Full size image This study reveals significant surface-wetting effects on NG-type LLT, which is induced by specific interactions (weak hydrogen bonding) between substrates and TPP molecules. This 'bottom-up' wetting mechanism of a microscopic nature is markedly different from the ordinary macroscopic mechanism responsible for wetting effects on phase separation, in which dispersion forces have a crucial role. We also demonstrate critical-point wetting, that is, a partial-to-complete wetting transition when approaching T SD . This critical-point wetting behaviour can be regarded as a strong evidence for the criticality associated with LLT. The interfacial tension between liquid I and II decreases in a manner consistent with the mean-field criticality [22] . This further supports the fact that the transition observed in TPP is truly 'LLT'. Contrary to the significant change in the kinetics for NG-type LLT, we reveal that SD-type LLT is not affected by surface-wetting effects, which can be explained by the non-conserved nature of the order parameter governing LLT. These findings may have a significant implication not only for the mechanism of LLT itself but also for applications of LLT. Our results show that we can use solid substrates or particles as a catalyst to promote LLT in a metastable region. This may open up novel possibilities not only for spatial patterning of liquid I and II using chemically or topologically patterned surfaces [4] , [10] but also for controlling the kinetics of LLT. The generality of the bottom-up wetting mechanism for LLT in atomic liquids, oxides and chalcogenides [16] is an interesting topic for future study. Samples Triphenyl phosphite is purchased from Acros Organics and used after extracting only a crystallizable part to remove impurities. We carefully avoided moisture to prevent chemical decomposition of TPP. We note that TPP molecules are known to decompose under the presence of water because of ester hydrolysis. A sample and a film were sandwiched between two cover glasses, the gap of which is determined by the thickness of the film. We observe the transformation process from liquid I to II near a quasi-1D interface between the liquid and the film from the top with phase-contrast microscopy (Olympus, BH2-UMA). Films (solid materials) used are as follows: PET (film thickness: 25 μm), poly(ethylene naphthalate) (25 μm), poly(imide) (25 μm), poly(vinylidene difluoride) (25 μm), PTFE (50 μm), PE (11 μm), gold (30 μm), platinum (20 μm), silver (30 μm) and aluminium (12 μm). Temperature was controlled within ±0.1 K by a computer-controlled hot stage (Linkam LK-600PH) equipped with a cooling unit (Linkam L-600A). Estimation of the Hamaker constant for dielectric substrates When the van der Waals force is the major interaction between liquid I, II and a solid surface, wettability should be estimated by a value of the Hamaker constant H [49] . H can be approximated as where ϵ I , ϵ II and ϵ s are the static dielectric constant of liquid I, II and the solid, respectively, ϵ I ( iν ), ϵ II ( iν ) and ϵ s ( iν ) are the dielectric function of liquid I, II and the solid evaluated at an imaginary frequency i ν, respectively, h is Plank's constant and ν 1 =2 πk B T / h =2.88×10 13 s −1 at 220 K. To estimate H , we need the dielectric functions of liquid I, II and the solid. Because it is difficult to obtain the dielectric function in the entire frequency range, we make the following two approximations: (i) The optical properties in a ultraviolet (UV) frequency range can be described as a single Lorentz oscillator: ϵ ( iν )=1+[( n 2 −1)/(1+ ν 2 + ν e 2 )] ( n : the refractive index of a material). (ii) The characteristic adsorption frequency in a UV frequency range, ν e , of liquid I, II and the solid is the same. We note that ν e values of liquid I and II are the same at least. Thus, the approximation is expected to be valid. We then obtain the following simple form of H [35] : where n I , n II and n s are the refractive indices of liquid I, II and the solid. Here, we use ν e =1.5×10 15 Hz [50] . From our dielectric measurements, the values of the static dielectric constants of liquid I and II at 220 K are estimated as 4.61 and 3.96, respectively. The refractive indices n of liquid I and II are then estimated, using the following Lorenz–Lorenz relation [51] : , where n is the refractive index, N 0 is the Avogadro number, ρ is the density, M is the molecular weight and α 0 is the electric polarizability. According to Cohen et al . [24] , the densities of liquid I and II are, respectively, 1.255 and 1.288 g cm −3 at 220 K. From the Lorentz–Lorentz relation, we estimated the refractive index of liquid I and II at 220 K as 1.634 and 1.655, respectively. To estimate the dielectric constant of a polar solid material, we used the Kirkwood-Frölich theory [51] . We neglect the temperature dependence of the refractive index, as the volume shrinkage of a solid substrate on cooling is negligible compared with that of liquids. We also estimated the refractive index of the TPP crystal from its dielectric constant by using the relation ϵ 0 = n 2 . For the estimation of H of calcium fluoride, we use the value of the UV absorption frequency of 3.8×10 15 Hz [35] . Estimation of the Hamaker constant for metallic substrates To estimate the dielectric constant of a metallic substrate, we use the Drude model [35] as the dielectric function of a metal: ϵ s ( iν )=1+[ ν p 2 /( ν 2 + νγ )]. We calculate H numerically by substituting equation (1), where ν p is the plasma frequency and γ is the damping frequency. Here we use the single Lorentz oscillator as the dielectric function for liquid I, II, as described in the previous section. We regard the static dielectric constant of all metals as infinity. The plasma frequency ν p and the damping frequency γ are estimated from literature [52] . How to cite this article: Murata K. & Tanaka H. Surface-wetting effects on the liquid–liquid transition of a single-component molecular liquid. Nat. Commun. 1:16 doi: 10.1038/ncomms1015 (2010).